Genomics of DNA cytosine methylation inEscherichia colireveals its role in stationary phase transcription DNA cytosine methylation regulates gene expression in mammals. In bacteria, its role in gene expression and genome architecture is less understood. Here we perform high-throughput sequencing of bisulfite-treated genomic DNA from Escherichia coli K12 to describe, for the first time, the extent of cytosine methylation of bacterial DNA at single-base resolution. Whereas most target sites (C m CWGG) are fully methylated in stationary phase cells, many sites with an extended CC m CWGG motif are only partially methylated in exponentially growing cells. We speculate that these partially methylated sites may be selected, as these are slightly correlated with the risk of spontaneous, non-synonymous conversion of methylated cytosines to thymines. Microarray analysis in a cytosine methylation-deficient mutant of E. coli shows increased expression of the stress response sigma factor RpoS and many of its targets in stationary phase. Thus, DNA cytosine methylation is a regulator of stationary phase gene expression in E. coli . DNA methylation at cytosines is an epigenetic mark that regulates gene expression and consequently major processes such as stem-cell development and cancer progression in higher eukaryotes [1] , [2] , [3] . In bacteria, methylation is best studied as part of restriction-modification (R-M) systems that have long been considered as contributing to bacterial immune response against incoming DNA including phages [4] . However, recent research has suggested that R-M systems may be 'selfish' elements that protect themselves against removal, through post-segregational killing of newly born progeny by pre-existing and stable restriction enzyme molecules [5] , [6] , [7] , [8] , [9] , [10] , [11] . In addition to being R-M components, methyltransferases are solitary (or orphan) enzymes that methylate DNA at specific sites, but are not associated with any restriction enzyme [12] . The best-studied solitary methyltransferase in E. coli is DNA adenine methyltransferase, which targets the G m ATC motif [13] . This methyl mark has important roles in regulating on-off gene expression by influencing the binding properties of transcription factors to DNA sites containing the methylated motif [14] , [15] ; it also influences replication by regulating the recruitment of the initiator of replication to the origin of replication [16] , [17] and regulates DNA repair by informing the methyl-directed mismatch repair system about the age of the DNA strand [18] , [19] , [20] . Another well-studied adenine methyltransferase is CcrM in Caulobacter crescentus , which methylates the GANTC site and acts as a cell cycle regulator [21] . A second DNA methyl transferase (Dcm) in E. coli methylates the internal cytosine in the CCWGG motif. Dcm is homologous to the methyltransferase that is part of the plasmid-encoded EcoRII R-M system, which also targets the CCWGG site [22] , [23] . Dcm confers resistance against parasitism by the EcoRII R-M system. This is because, in the presence of a functional Dcm, Eco RII-target sites will be kept methylated even when the R-M system is disturbed, thus preventing post-segregational killing [24] . To our knowledge, this, an association between Dcm and Tn3 transposition [25] , and lambda DNA recombination [26] , and a very recently discovered role in regulating ribosomal gene expression in stationary phase [27] , remain the only phenotypes associated with Dcm. Despite having been identified in the 1970s [28] and cloned in the 1980s [29] , Dcm remains poorly studied. Low-resolution genome-scale studies have shown that not all target sites of Dcm (and DNA adenine methyltransferase) are methylated in-vivo [30] , confirming previous work by Bhagwat and colleagues [31] . However, the low resolution of the above studies precluded careful genome-scale analysis of partially methylated and unmethylated sites. Though regulation of gene expression by cytosine methylation has been described for mammals [3] , such results in bacteria have been limited largely to adenine methylation with little information on its cytosine counterpart. Here, we present the first single-base-resolution genome-scale study of cytosine methylation in E. coli . We first perform high-throughput sequencing of bisulfite-treated genomic DNA [32] from E. coli K12, thus quantifying the extent of cytosine methylation at single-base resolution across various phases of batch culture. We unveil patterns of methylation that might be consistent with reducing the risk of non-synonymous m C->T transitions. We also perform microarray analysis of gene expression in a Δ dcm strain of E. coli , thus identifying a role for methylation in controlling gene expression levels during stationary phase. Occurrence of the CCWGG motif The E. coli K12 MG1655 genome contains 24,090 instances of the CCWGG motif (on either strand; 12,045 on each strand), which is targeted by the Dcm DNA cytosine methyltransferase. This is ~27% more than the expected by random chance, given the genome's overall A/T content [33] . This is difficult to interpret; however, this 27% increase over expectation is less dramatic than in organisms such as Pseudomonas aeruginosa , where the occurrence of CCWGG motif is more than double the expected value ( http://tools.neb.com/~vincze/cutfreq/CCWGG.html ). Unlike the GATC motif in which the adenine is methylated [34] , [35] , the occurrence of CCWGG motif is not strongly constrained or particularly over-represented in genes or regulatory genes: ~93% of these motifs are located within genes, which is consistent with the genomic average considering the relative sizes and difference in A/T content between genes and intergenic regions. The number of CCWGG motifs in a gene correlates with its length ( ρ =0.75 Pearson Correlation; Fig. 1a ). The frequency of occurrence of the CCWGG motif per kilobase of sequence follows a Poisson distribution, with an average of 2.6 occurrences of the motif on each strand; this is as expected by random chance, given the total number of CCWGG motifs in the entire genome ( Fig. 1b,c ). 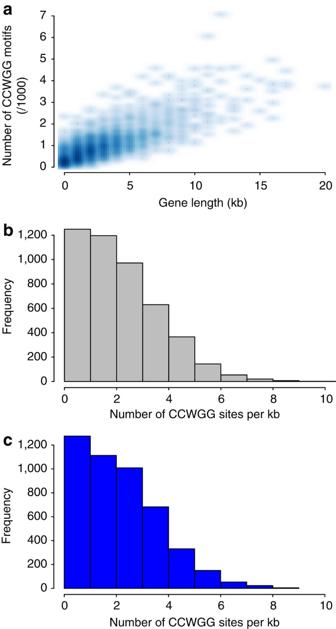Figure 1: Occurrence of the CCWGG motif. (a) Smooth scatter plot showing the correlation between the number of CCWGG motifs per gene (yaxis) and the length of the gene in which motif occurrence is computed (xaxis). (b) Histogram showing the null hypothesis that the occurrence of the CCWGG motif per kilobase of DNA sequence should follow a Poisson distribution withλ=2.6 (total number of CCWGG motifs×1000 per genome size) (c) Histogram showing the distribution of the numbers of CCWGG motifs found per kb of genomic sequence. Figure 1: Occurrence of the CCWGG motif. ( a ) Smooth scatter plot showing the correlation between the number of CCWGG motifs per gene ( y axis) and the length of the gene in which motif occurrence is computed ( x axis). ( b ) Histogram showing the null hypothesis that the occurrence of the CCWGG motif per kilobase of DNA sequence should follow a Poisson distribution with λ =2.6 (total number of CCWGG motifs×1000 per genome size) ( c ) Histogram showing the distribution of the numbers of CCWGG motifs found per kb of genomic sequence. Full size image Bisulfite sequencing of E. coli genomic DNA To identify cytosines that are methylated in E. coli K12 MG1655, we first isolated genomic DNA from cultures grown in batch to mid-exponential, late-exponential, transition-to-stationary and stationary phases. We then treated the DNA with a commercial bisulfite reagent that converts unmethylated cytosines to uracil, but leaves methylated residues unaffected, and produces single-stranded DNA. Following synthesis of the second strand of DNA, we carried out multiplexed DNA sequencing on an Illumina GA IIx system producing several million 36-mer reads ( Supplementary Table S1 ). Our data provide a ~20-fold coverage of the E. coli genome per sample. Using Bismark software [36] , we mapped fully bisulfite-converted forward and reverse read (C->T and G->A conversions of the forward strand) to similarly converted versions of the reference genome; the best of the four possible alignments was compared with the normal reference sequence to enable calls on the methylation state of all cytosine positions in the read. To our knowledge, this is the first genome-wide base-resolution study of cytosine methylation in any bacterium. To assess the quality of our methylation calls, we performed similar experiments on an otherwise isogenic Δ dcm mutant strain. The bisulfite reagent used has a 99% conversion rate; given this and the assumption that dcm is the only gene encoding a DNA cytosine methyltransferase in E. coli , we should expect ~1% of cytosines in the Δ dcm experiment to be called methylated. Across the four Δ dcm samples, <1.5% (range: 1.33–1.57%) of cytosines are called as methylated, showing that our data are reliable. Every cytosine is covered by multiple reads each with its own methylation call. This allows us to calculate, for each cytosine, the fraction of mapped reads determined to be methylated, which we define as the 'extent of methylation' ratio ( R met ). Using our stationary phase sample, where the population is least dynamic in terms of DNA replication, we first identified cytosines where every mapped read is defined as methylated ( R met =1). We then used the sequences surrounding the methylated cytosine and identified sequence motifs, which recovered the known target site for Dcm (CCWGG, where W stands for A or T; Fig. 2a ) [12] . In stationary phase cells, almost all reads mapping to CCWGG sites were called methylated (mean R met =0.98). On the other hand, only sporadic cases of methylated reads mapping to non-CCWGG sites were observed (mean R met =0.02; Supplementary Fig. S1 ). A similar difference is observed for R met values at CCWGG motifs between the wildtype and Δ dcm ( Fig. 2b ). 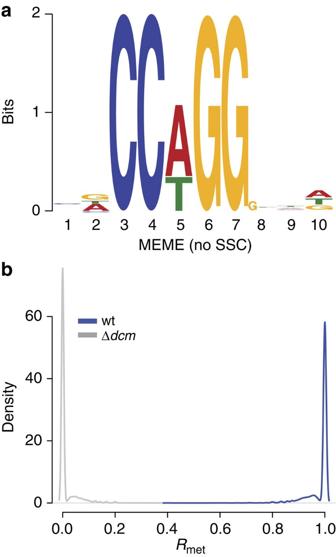Figure 2: Bisulfite sequencing ofE. coligenomic DNA: basic information. (a) Sequence motif surrounding the cytosine methylated by Dcm in stationary phase cells ofE. coliK12 MG1655. (b) Probability density function (as determined using Kernel density estimation implemented inR) ofRmetvalues for the internal cytosine at C(m)CWGG sequences obtained during stationary phase for the wild-type (blue) and Δdcmstrains ofE. coli. Figure 2: Bisulfite sequencing of E. coli genomic DNA: basic information. ( a ) Sequence motif surrounding the cytosine methylated by Dcm in stationary phase cells of E. coli K12 MG1655. ( b ) Probability density function (as determined using Kernel density estimation implemented in R ) of R met values for the internal cytosine at C (m) CWGG sequences obtained during stationary phase for the wild-type (blue) and Δ dcm strains of E. coli . Full size image In summary, these results reassert that methylation occurs exclusively at CCWGG; show that during stationary phase methylation of CCWGG sites is nearly complete; and demonstrate that Dcm is the only cytosine methyltransferase in the E. coli strain used here (based on data obtained from the Δ dcm strain). Cytosine methylation and gene expression in E. coli Cytosine methylation is a key regulator of gene expression in mammals, with major influence on processes such as development and cancer progression. In bacteria, however, DNA adenine methylation has been recognized as a regulator of gene expression, primarily by influencing the activities of transcription factors whose effects are correlated with the target's methylation status [14] , [15] . However, until very recently [27] when cytosine methylation was shown to regulate ribosomal gene expression in stationary phase, no role for cytosine methylation in gene expression control had been documented for bacteria, at least for enterobacteria. Despite the widespread and apparently 'random' occurrence of the CCWGG motif, a recent study has shown that where present in intergenic regions, several CCWGG sites are clustered together [27] , thus leading to immediate speculation on the role of methylation in gene regulation. However, our analysis of the occurrence of the CCWGG motif across 2,558 experimentally verified transcription factor-binding sites in the RegulonDB database [37] showed that this motif occurs only 69 times in these sequences, which is not significantly different from the trend in the rest of the genome. Further, only two of these transcription factor-binding sequences contained more than one CCWGG motif. This is unlike results obtained with the GATC motif, in which the adenine is methylated, and which is over-represented in CRP-binding loci [34] . Thus, analysis of the genome sequence alone provides little statistical evidence that cytosine methylation influences gene expression on a global scale by interfering with transcription factor-DNA interactions. To experimentally investigate the role of cytosine methylation in gene expression in E. coli on a genomic scale, we performed microarray analysis of gene expression in the wild-type and Δ dcm strains of E. coli K12 MG1655 ( Fig. 3a ), thus identifying genes that are differentially expressed in Δ dcm during mid-exponential, late-exponential, transition-to-stationary and stationary phases of batch growth. As there is little cytosine methylation in Δ dcm , gene expression changes identified here are directly or indirectly caused by the absence of cytosine methylation. 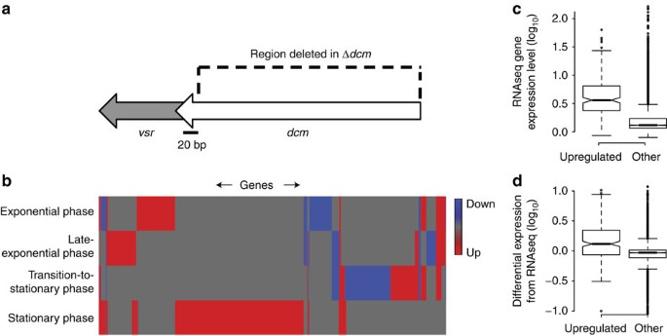Figure 3: Effect of Δdcmon gene expression inE. coli. (a) A schematic diagram showing thedcmlocus and the region deleted in this study. In the Δdcmstrain, 1250 bp ofdcmwere deleted (from 4 to 1254), leaving 165 bp at the 3′ end of the gene. This leaves 145 bp upstream of the start codon ofvsr, to ensure the expression ofvsrwas not affected. (b) Heat map showing differential expression (binary coding: red for upregulation, blue for downregulation, grey for no significant differential expression) of genes in Δdcmwhen compared with the wildtype during exponential, late-exponential, transition-to-stationary and stationary phases of batch culture. Genes are grouped together by hierarchical clustering using Euclidean distance. (c) Boxplot showing wildtype expression levels on theyaxis (number of reads mapping per base for each gene, normalized by the total number of reads obtained in the sequencing experiment; all values were uniformly multiplied by 107and log transformed) of genes that are upregulated in Δdcmduring stationary phase, compared with a control set of all other genes (referred to as 'other') (d) As inc, except that this panel shows the fold change in expression between stationary and exponential phases of growth in the wildtype. In the boxplots, the boxes cover the interquartile range (IQR) between the first and the third quartiles (Q1 and Q3, respectively); the whiskers are drawn at the extreme value that is no more than Q3+1.5×IQR, and no less than Q1−1.5×IQR. Incandd, theyaxis is terminated at the marked extremes for effective visualization. Figure 3: Effect of Δ dcm on gene expression in E. coli . ( a ) A schematic diagram showing the dcm locus and the region deleted in this study. In the Δ dcm strain, 1250 bp of dcm were deleted (from 4 to 1254), leaving 165 bp at the 3′ end of the gene. This leaves 145 bp upstream of the start codon of vsr , to ensure the expression of vsr was not affected. ( b ) Heat map showing differential expression (binary coding: red for upregulation, blue for downregulation, grey for no significant differential expression) of genes in Δ dcm when compared with the wildtype during exponential, late-exponential, transition-to-stationary and stationary phases of batch culture. Genes are grouped together by hierarchical clustering using Euclidean distance. ( c ) Boxplot showing wildtype expression levels on the y axis (number of reads mapping per base for each gene, normalized by the total number of reads obtained in the sequencing experiment; all values were uniformly multiplied by 10 7 and log transformed) of genes that are upregulated in Δ dcm during stationary phase, compared with a control set of all other genes (referred to as 'other') ( d ) As in c , except that this panel shows the fold change in expression between stationary and exponential phases of growth in the wildtype. In the boxplots, the boxes cover the interquartile range (IQR) between the first and the third quartiles (Q1 and Q3, respectively); the whiskers are drawn at the extreme value that is no more than Q3+1.5×IQR, and no less than Q1−1.5×IQR. In c and d , the y axis is terminated at the marked extremes for effective visualization. Full size image Across the four conditions tested, 510 genes are differentially expressed in Δ dcm when compared with the wildtype; of these, 362 are only upregulated, 137 downregulated and the remaining few are upregulated in one condition and downregulated in another. There is no global statistical association between the occurrence of a CCWGG motif in gene-upstream regions or the gene body and differential expression (with differentially expressed and other genes showing similar densities of CCWGG motifs of 2.7–2.9 motifs per kb of gene sequence); nevertheless, it must be noted that this does not rule out any direct role of CCWGG motifs in controlling proximal gene expression at specific loci. Finally, largely distinct sets of genes are differentially expressed in different time points ( Fig. 3b ). Here, we describe selected trends observed in our analysis of these microarray data. Effect of Δ dcm on stationary phase gene expression Of the 362 genes that are upregulated (in Δ dcm when compared to the wildtype) in at least one of the four conditions tested, 222 (61%) do so in stationary phase. In contrast to other phases of growth where comparable numbers of genes are up- or downregulated, very few (three) genes are downregulated in stationary phase ( Fig. 3b ). In agreement with a recent work [27] , 15 genes involved in translation and ribosomal biogenesis (as defined by the COG database) are upregulated in Δ dcm . Further analysis of the wild-type expression levels of genes that are upregulated in stationary phase showed the following: these are expressed at higher levels than other genes during stationary phase in wildtype cells ( P <10 −6 ; Wilcoxon test; Fig. 3c ); show higher fold change in expression levels between stationary and exponential phases in the wild-type strain ( P <10 −6 ; Wilcoxon test; Fig. 3d ); and are targets of RpoS (the stationary phase sigma factor) identified by Weber and colleagues [38] (37 genes; P =9.1×10 −6 ; Fisher test compared with genes upregulated in other phases of growth). Note that difficulties in normalization of microarray data between exponential and stationary phase (as previously discussed by others [39] ) made us use data obtained from RNA-seq experiments [40] to perform the calculations on wild-type gene expression described above; though similar issues may be valid even for RNA-seq data, these should not substantially alter our qualitative conclusions. In summary, in Δ dcm , genes that seem to be already stationary phase-specific in wild-type cells are further upregulated. We observe that several members of the RNA polymerase complex are upregulated in Δ dcm during stationary phase; this is particularly true for rpoS , which we were able to validate using RT–PCR and western blots ( Table 1 ; Supplementary Fig. S2 ). We suspect that much of the general transcriptional upregulation observed in stationary phase Δ dcm cells is an indirect consequence of the upregulation of RpoS. However, this does not affect the culture's long-term viability during stationary phase in batch culture ( Supplementary Fig. S3 ). Table 1 Gene expression change of selected genes in Δ dcm in comparison to the wildtype. Full size table It is notable that there are five CCWGG motifs present in the rpoS promoter and gene body. The first is ~95 bp upstream of the transcription start site (TSS), the second ~140 bp downstream of the TSS and the third ~47 bp upstream of the ORF; the other two are further downstream in the ORF. Of these, there is a dramatic increase in R met value from 0.2 to 1.0 from exponential to stationary phase for one motif, present ~370 bp downstream of the ORF start site. There is a weaker increase, from 0.83 to 1.0 and 0.76 to 1.0, respectively, for the first two sites above that are closest to the TSS. Whether any of these have a direct role in regulating rpoS expression by interfering with transcription factor binding is not known and remains to be investigated; however, none of these sites overlap with known CRP or ArcA-binding sites, with the first site being closest, lying ~25 bp upstream of a CRP-binding site. In wild-type cells, 256 genes are differentially expressed between mid- and late-exponential phase populations; in Δ dcm , there is an ~1.9-fold increase in the number of differentially expressed genes (488) between the two phases. Two-thirds of the 256 genes with variable expression in the wildtype are included in the considerably larger list of those that change in expression in Δ dcm . Among the genes differentially expressed only in Δ dcm are 45 genes involved in ribosomal biogenesis and translation ( P <10 −6 ; Fisher's exact test), most of which are upregulated in late-exponential phase. This, we suggest, precedes the enhanced gene expression of ribosomal genes observable in stationary phase [27] . Upregulation of lamB in Δ dcm during mid-exponential phase During mid-exponential phase, 85 genes are upregulated in Δ dcm when compared to the wildtype. Among these is lamB , which displays a 3-fold upregulation in our microarray data (>4.5-fold upregulation in RT–PCR validation, ΔΔ Ct=2.2), along with malK , another gene encoded in the same operon ( Table 1 ). LamB is a maltoporin, whose functions include being a receptor for lambda phage [41] . The presence of DNA cytosine methylation might have a role in minimizing the possibility of phage infection in mid-exponential phase E. coli populations where rapid growth is a trigger for lytic explosions. Partial methylation of CCWGG sites in mid-exponential phase To assess the differences between different stages of batch growth in the extent of methylation of cytosines, we used our bisulfite-sequencing data to calculate R met for the internal cytosine in each CCWGG motif with at least five mapped reads (~89% of all CCWGG motifs across the four conditions combined). Across the four time-points, an average R met of 0.91 (median=1.00) was observed; however, the value increased from 0.80 (median=0.85) for mid-exponential phase sample to 0.98 (median=1.00) for the stationary phase sample in a progressive fashion ( Figs 4a and 5a ). This shows that there are many Dcm-target sites in the genome, which are methylated only in a fraction of the population of mid-exponential phase E. coli DNA. 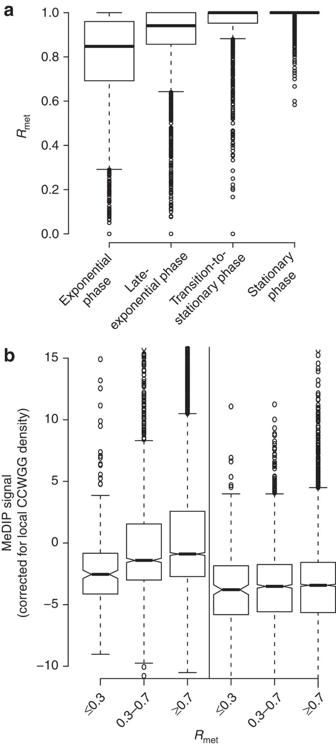Figure 4: Growth phase and extent of methylation. (a) Boxplots showing the distributions ofRmetvalues obtained during exponential, late-exponential, transition-to-stationary and stationary phases of a batch culture of wild-typeE. coliK12 MG1655. (b) MeDIP signal (normalized by LOESS against the local density of CCWGG motifs) for C(m)CWGG sites with low, medium and highRmetvalues; the left panel is for the wildtype, whereas the right panel shows MeDIP experiments performed in the Δdcmstrain. A description of the quantity used to measure MeDIP signal is given inSupplementary Fig. S4. In the boxplots, the boxes cover the interquartile range (IQR) between the first and the third quartiles (Q1 and Q3, respectively); the whiskers are drawn at the extreme value that is no more than Q3+1.5×IQR, and no less than Q1−1.5×IQR. Inb, theyaxis is terminated to −10≤y≤15 for effective visualization. Figure 4: Growth phase and extent of methylation. ( a ) Boxplots showing the distributions of R met values obtained during exponential, late-exponential, transition-to-stationary and stationary phases of a batch culture of wild-type E. coli K12 MG1655. ( b ) MeDIP signal (normalized by LOESS against the local density of CCWGG motifs) for C (m) CWGG sites with low, medium and high R met values; the left panel is for the wildtype, whereas the right panel shows MeDIP experiments performed in the Δ dcm strain. A description of the quantity used to measure MeDIP signal is given in Supplementary Fig. S4 . In the boxplots, the boxes cover the interquartile range (IQR) between the first and the third quartiles (Q1 and Q3, respectively); the whiskers are drawn at the extreme value that is no more than Q3+1.5×IQR, and no less than Q1−1.5×IQR. In b , the y axis is terminated to −10≤y≤15 for effective visualization. 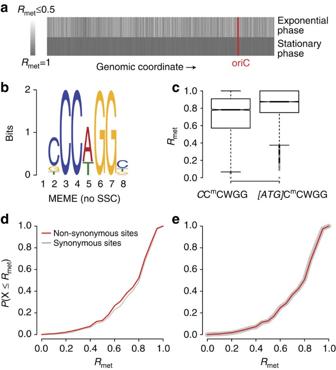Figure 5: Genomic correlates of partial methylation. (a) Heatmap showingRmetvalues for C(m)CWGG motifs along the chromosome ofE. coliK12 MG1655 during exponential and stationary phases of batch culture. Grey stands forRmet=1, whereas white representsRmet<=0.5. The red vertical line approximately marks the origin of replication. (b) Sequence motif obtained for sequences withRmet<=0.2 during exponential phase. (c) Boxplots showing the distribution ofRmetvalues for [ATG]C(m)CWGG and CC(m)CWGG motifs during exponential phase. The boxes cover the interquartile range (IQR) between the first and the third quartiles (Q1 and Q3, respectively); the whiskers are drawn at the extreme value that is no more than Q3+1.5×IQR, and no less than Q1−1.5×IQR. (d) Cumulative distribution ofRmetvalues for C(m)CWGG sequences, where the internal cytosine is positioned at synonymous (grey) and non-synonymous (red) locations. (e) As ind, except that the assignment ofRmetvalues to specific cytosine positions was randomized. Full size image Figure 5: Genomic correlates of partial methylation. ( a ) Heatmap showing R met values for C (m) CWGG motifs along the chromosome of E. coli K12 MG1655 during exponential and stationary phases of batch culture. Grey stands for R met =1, whereas white represents R met <=0.5. The red vertical line approximately marks the origin of replication. ( b ) Sequence motif obtained for sequences with R met <=0.2 during exponential phase. ( c ) Boxplots showing the distribution of R met values for [ATG]C (m) CWGG and CC (m) CWGG motifs during exponential phase. The boxes cover the interquartile range (IQR) between the first and the third quartiles (Q1 and Q3, respectively); the whiskers are drawn at the extreme value that is no more than Q3+1.5×IQR, and no less than Q1−1.5×IQR. ( d ) Cumulative distribution of R met values for C (m) CWGG sequences, where the internal cytosine is positioned at synonymous (grey) and non-synonymous (red) locations. ( e ) As in d , except that the assignment of R met values to specific cytosine positions was randomized. Full size image To test the reliability of this observation, we also performed methylated-DNA immunoprecipitation (MeDIP)-seq experiments [42] , in which immunoprecipitated fragments of the chromosome containing methylated cytosines were subjected to high-throughput sequencing ( Supplementary Fig. S4 and Supplementary Table S2 ). We find that regions determined by our bisulfite-sequencing experiment to be partially methylated in mid-exponential phase have weaker MeDIP signals than those that are fully methylated ( Fig. 4b ; P <10 −6 , Wilcoxon test comparing the MeDIP signals for sites with R met <=0.3 and those with R met >=0.7). This is despite the considerably poorer resolution of the MeDIP approach and the fact that signals are dependent on the clustering of methylated cytosines. A trivial explanation for the reduced level of methylation in the exponential phase sample is the presence of newly synthesized DNA, which is yet to be methylated. In rapidly dividing E. coli cells, multiple rounds of replication get initiated between any pair of adjacent division events. Consequently, such cells will have more copies of the region of the chromosome around the origin of replication than near the terminus. This is observed in our data, which, without considering methylation calls, is equivalent to that from a quantitative genome-sequencing experiment ( Supplementary Fig. S5 ). In the exponential phase sample, more reads map to the region around the origin than around the terminus; this, however, is not the case in the stationary phase sample. However, sites of partial methylation are not substantially concentrated around the origin or regions of the chromosome with new DNA to the extent detectable in non-synchronized mixed populations ( Fig. 5a ; Supplementary Fig. S6 ). In fact, partially methylated sites are distributed across the chromosome. This implies the existence of non-trivial explanations for the occurrence of partially methylated CCWGG sites in the genome. This is further substantiated by the observation that two independent biological samples, one processed by bisulfite sequencing and the other by MeDIP-seq, give consistent results. To identify specific signals associated with partial methylation, we performed a motif search using sequences surrounding CCWGG sites with R met ≤0.2 in mid-exponential phase [43] . We observe an extended motif C C (m) CWGG at these sites ( Fig. 5b ). We then compared the R met values for all CCCWGG and [ATG]CCWGG motifs in the genome and found that the extent of methylation is significantly less in the former (mean R met =0.72) than in the latter (mean R met =0.83; P <10 −6 , Wilcoxon test; Fig. 5c ). Finally, we analysed the positioning of partially methylated cytosines to speculate on the possibility that these sites may be selected. We based this analysis on the foundation that methylated cytosines are mutation hotspots because of their tendency to get deaminated to form thymines [44] . Though E. coli encodes a very short-patch repair (VSR) system to correct such mutations [45] , [46] , [47] , it is expressed and active only during stationary phase. We classified all C C WGG cytosines located within genes into those that, if mutated in a methylation-dependent fashion, would lead to synonymous or non-synonymous changes. This classification was based purely on their ability to change the amino acid (including non-sense mutations that introduce a stop codon) encoded by the respective codon, and did not include other subtle effects such as changing mRNA stability or influence on protein–DNA interactions. First, we find that the 'methylatable' cytosine in a significantly higher proportion of C CCWGG motifs (~60%) is located at non-synonymous sites, when compared to [ATG]CCWGG sites (~54%; P <10 −6 ; Fisher exact test). Next, using our bisulfite-sequencing data, we tested the association between the extent of methylation (in mid-exponential phase) and the tendency of a particular cytosine to be positioned in synonymous or non-synonymous locations. We find a statistically significant difference between partially and fully methylated cytosines in their tendency to be located at synonymous or non-synonymous positions. Whereas ~60% of C C WGG cytosines with R met ≤0.5 (67% for R met ≤0.2) are located at non-synonymous sites, only ~51% of those with R met ≥0.9 are so located ( P =4×10 −6 ; Fisher exact test). In general, there is a slight, yet statistically significant, difference between the distributions of R met values for synonymous and non-synonymous sites ( P =2×10 −5 ; Kolmogorov–Smirnov test; Fig. 5d,e ; Supplementary Fig. S7 ). In summary, we speculate that during exponential phase when multiple rounds of replication occur in the absence of the VSR repair system, cytosine methylation by Dcm is probably slowed down, particularly at non-synonymous sites, potentially as a consequence of the presence of the extended CCCWGG motif. This might be consistent with the hypothesis that partial methylation might reduce the risk of mutation; however, the strength of the signals observed here suggests that it is likely to be a relatively minor effector. In this study, we performed high-throughput sequencing of bisulfite-treated genomic DNA from E. coli K12 grown to mid-exponential, late-exponential, transition-to-stationary and stationary phases of growth, to identify its methylation status. Whereas most CCWGG sites are fully methylated in stationary phase cells, there is a progressive increase in the extent of methylation from exponential to stationary phase. Partial methylation in mid-exponential phase cells is associated with the presence of the extended CCCWGG motif, and has a slight tendency to be localized to non-synonymous sites. Methylated cytosine is a mutational hotspot that can spontaneously convert to thymine at a rate of 5.8×10 −13 per second [48] ; the rate is three orders of magnitude higher in single-stranded DNA, a state that would occur during replication and transcription. Though E. coli has a VSR system to reduce such mutations, it is not expressed during exponential phase by a post-transcriptional mechanism [45] , [46] , [47] . We speculate here that sites for partial methylation are selected to reduce the slight risk of potentially deleterious non-synonymous mutations; this happens especially in exponential phase when numerous new progeny are created and the VSR system is not expressed. The possible products of methylation-dependent mutations, namely the C[C/T]W[A/G]G sites, are severely under-represented (at ~25% of the expected levels) in the E. coli genome. It has been argued that VSR replacing normal CTWGG sites to CCWGG might have caused depletion of the former and the enrichment of the latter [49] . An alternative argument is that this might be a mechanism to ensure that the VSR system can efficiently detect and correct mutant sites with minimal confusion arising from 'normal' C[C/T]W[G/A]G sites; there might be an interplay of both forces in determining the final oligonucleotide usage in the E. coli genome. However, several other organisms might, in fact, make use of cytosine methylation to generate genotypic diversity during stationary phase; for example, Vibrio cholerae encodes a Dcm (targeting the external cytosine in RCCGGY motif), but not a VSR repair system [50] . Analysis of the genome of V. cholerae shows that a striking 97% of 'methylatable' cytosines are at non-synonymous positions, suggesting a strong preference for having methyl-dependent mutations at non-synonymous sites (3,964 of 4,074 sites on either strand of both chromosomes). Contrary to the situation in mammals, a role for methylation in the control of gene expression in bacteria has been limited to N6-adenine methylation. Using microarrays, we show upregulation of genes in Δ dcm —in comparison to the wildtype—during stationary phase. Much of this does not represent any reorganization of the transcriptional state, but instead increased expression of genes that are already stationary-phase specific. This might be caused by the increased expression of RpoS, which we observe in our microarrays and validate using RT–PCR and western blots. Thus, our study includes Dcm as a possible regulator of rpoS expression. This is in addition to the recently discovered role of Dcm in controlling ribosomal gene expression during stationary phase [27] ; we suggest that the expression of these genes begins to increase in late-exponential phase. Does the increased stationary phase gene expression have any consequence to E. coli fitness under laboratory conditions? No difference can be observed between the wildtype and Δ dcm strains in their long-term stationary phase survival during batch culture in Luria–Bertani medium. However, this does not rule out specific fitness defects in Δ dcm in complex natural environments, where E. coli might be spending much of its time in stationary phase, with an estimated doubling time of 40 h [51] . In addition, we reveal increased expression of lamB , which encodes a maltoporin that is also the receptor for lambda phage, during mid-exponential phase in Δ dcm . Thus, Dcm might have a role in reducing susceptibility of E. coli to lytic infections by lambda phage. In fact, it has been previously shown that unmethylated lambda DNA is more recombinogenic than methylated DNA, thus establishing a link, albeit at a level different to that implied by our gene expression analysis [26] , between cytosine methylation and phage infection. The mechanism by which Dcm/cytosine methylation affects gene expression in E. coli is not known. It is not known whether there are any DNA-binding proteins in E. coli with transcriptional regulatory roles whose activities are dependent on the methylation state of the substrate DNA. However, cytosine methylation also alters the mechanical properties of DNA [52] , and this might have profound consequences on transcription. In summary, we suggest that cytosine methylation might have a role in determining aspects of a bacterium's genome structure and may also be a regulator of transcription, especially during the stationary phase. Strains and general growth conditions The E. coli K12 MG1655 bacterial strains used in this work are the wildtype (F- lambda- ilvG- rfb-50 rph-1) and Δ dcm ( Fig. 3a ). Luria–Bertani (0.5% NaCl) broth and agar (15 g l −1 ) were used for routine growth. Where needed, ampicillin, kanamycin and chloramphenicol were used at final concentrations of 100, 30 and 30 μg ml −1 , respectively. Construction of E. coli MG1655 knock-outs Disruption of dcm in the E. coli chromosome was achieved by the λ Red recombination system, previously described by Datsenko and Wanner [53] . Primers designed for this purpose are P4: 5′-TTAACCTGTCGGCCATCTCAGATGGCCGGTGAAATCTATGATTCCGGGGATCCGTCGACC-3′ and P1: 5′-ATAGGCCTGAGTGTCCGAAACCGGAATACGGAATTTCGCTGTGTAGGCTGGAGCTGCTTC-3′. Sets of additional external primers were used to verify the correct integration of the PCR fragment by homologous recombination ( Forward : 5′-GTCGATCACAAGGTGATAG-3′; Reverse : 5′-GCAGCGATATTCATCAACG-3′). RNA extraction and microarrays procedures RNA was extracted using Trizol reagent (Invitrogen) and mirVana miRNA isolation kit (Ambion) as reported previously [40] . Briefly, cells pelleted by centrifugation (10,000 g , 10 min, 4 °C) were stored at −80 °C until required. RNA was isolated using Trizol (Invitrogen) following the manufacturer's protocol until the chloroform extraction step. The aqueous phase was placed in columns from the mirVana miRNA isolation kit (Ambion) and washed following the manufacturer's protocol. Finally, the total RNA was eluted in 50 μl of RNase-free water. The concentration was then determined using a Nanodrop ND-1000 machine (NanoDrop Technologies), and RNA quality was tested by visualization on agarose gels and by Agilent 2100 Bioanalyser (Agilent Technologies, Palo Alto, CA, USA). For the generation of fluorescence-labelled cDNA, we used the FairPlay III Microarray Labelling Kit (Stratagene) as described previously [40] . Briefly, 1 μg of total RNA was subjected to cDNA synthesis in a reverse transcription reaction using random primers. The amino allyl labelled cDNA (at dUTP) thus obtained was coupled to a Cy3 dye (GE Healthcare) containing a NHS-ester leaving group. The labelled (Cy3) cDNA was hybridized to the probe DNA on microarrays by incubating at 65 °C for 16 h. The unhybridized labelled cDNA was removed and the hybridized labelled cDNA was visualized using an Agilent Microarray Scanner. RT–PCR for validation To validate the results of the microarray analysis, quantitative reverse transcriptase PCR was carried out using specific primers to the mRNA targets showing up- or downregulation, and control targets not showing differential expression. RNA was extracted as described above from wild-type and Δ dcm cells, and 30 ng total RNA was used with the Express One-Step SYBR GreenER kit (Invitrogen) according to the manufacturer's guidelines, using a MJ Mini thermal cycler (Bio-Rad). All primers and results are listed in Supplementary Tables S3 and S4 , respectively. Bisulfite conversion Wildtype E. coli K12 MG1655 and Δ dcm cells were grown to the desired OD and the genomic DNA extracted using a Wizard Genomic DNA purification kit (Promega). The DNA was sheared to ~2 kb using a Bioruptor (Diagenode). Bisulfite conversion was performed using the EpiTect Bisulfite kit (Qiagen), following the manufacturer's guidelines on 'Sodium Bisulfite Conversion of Unmethylated Cytosines in Small Amounts of Fragmented DNA'. Single-stranded DNA resulting from the BS conversion was converted to double-stranded DNA using random primers (Invitrogen). The DNA was then further sheared to approximately 200 bp fragments, before proceeding with the library construction. Library construction and Solexa sequencing Prior and post library construction, the concentration of DNA was measured using the Qubit HS DNA kit (Invitrogen). Library construction was done using the ChIP-Seq Sample Prep kit with customized barcoded adapters adopted from Lefrancois et al . [54] , to allow multiplexing of eight samples. Samples were loaded at a concentration of 10 pM. Public data sources The E. coli K12 MG1655 genome and gene coordinate annotations were downloaded from the KEGG database [55] . A list of 140 genes regulated by RpoS were obtained from Weber et al [38] . RNA-seq data for stationary and mid-exponential phase [40] were generated in our lab as reported previously and RPKM [56] values obtained from this were used. Analysis of genomic data Barcoded reads obtained from Illumina Genome Analyzer IIx were first assigned to their respective samples. Subsequently, methylation calls were made using Bismark software [36] , which makes use of Bowtie [57] for read-to-genome mapping. Sequence motifs were identified using the MEME software [43] . Gene expression analyses were performed on a previously described custom-designed isothermal Agilent microarray platform, and analysed as described earlier [40] . Briefly, array data were background corrected using normexp [58] and normalization performed using VSN [59] . Differential expression in the deletion strains compared with the wild-type was called at FDR-adjusted P -value of 0.05, and a fold-change of at least two. To reduce the false-positive rates, a second round of analysis was performed, in which each gene was represented by the average expression value across all probes that map to it. The above procedure for processing and calling differential expression was adopted again. Finally, genes called as differentially expressed as per both the above analysis pipelines were used and discussed in this study. All statistical tests were carried out using R ( http://r-project.org ). Acccession codes: Bisulfite sequencing and MeDIP-seq data have been deposited in the NCBI Sequence Read Archive under accession codes SRX116370 and SRX118253 , respectively. Microarray data have been deposited in Array Express under accession code E-MEXP-3569 . How to cite this article: Kahramanoglou C, et al . Genomics of DNA cytosine methylation in Escherichia coli reveals its role in stationary phase transcription. Nat. Comm. 3:886 doi: 10.1038/ncomms1878 (2012).